Genetic dissection of axon regeneration viain vivoelectroporation of adult mouse sensory neurons Manipulating gene expression in vivo specifically in neurons with precise spatiotemporal control is important to study the function of genes or pathways in the nervous system. Although various transgenic approaches or virus-mediated transfection methods are available, they are time consuming and/or lack precise temporal control. Here we introduce an efficient electroporation approach to transfect adult dorsal root ganglion (DRG) neurons in vivo that enables manipulation of gene expression in an acute and precise manner. We have applied this method to manipulate gene expression in three widely used in vivo models of axon injury and regeneration, including dorsal column transection, dorsal root rhizotomy and peripheral axotomy. By electroporating DRGs with small interfering RNAs against c-jun to specifically deplete c-Jun in adult neurons, we provide evidence for the role of c-Jun in regulation of in vivo axon regeneration. This method will serve as a powerful tool to genetically dissect axon regeneration in vivo . Manipulation of gene expression via transgenic technology has been a valuable tool for studying the role of a particular gene(s) or pathway(s) in the nervous system in vivo , especially during development. However, the genetic studies of the adult nervous system have been lagged behind due to difficulties in manipulating gene expression, specifically in adult neurons. For genes that have important roles in development, traditional knockout approach, in many cases, results in either early embryonic lethality or compensatory responses, both of which confound the study of gene functions in adult animals. Although the inducible knockout approach using the Cre recombinase can solve some of these problems, generating conditional knockout mice is an expensive and highly time-consuming process. Acute virus-based gene delivery is another way of genetic manipulation in adult neurons that allows precise spatiotemporal control. However, it involves labour-intensive processes, such as production and purification of viral particles for each gene of interest. In addition, many viral vectors could activate the immune system of the host, which might also affect the experimental results and interpretation. Electroporation is a rapid and effective method of gene delivery, and in utero electroporation has recently emerged to be an important tool in studying neurodevelopment in vivo [1] . This approach is moving forward and a recent study has successfully transfected adult neural progenitors using in vivo electroporation [2] . The dorsal root ganglia (DRG) contain a diverse group of sensory neurons that convey different sensory stimuli, such as pain, temperature, touch and body posture, to the brain. Each DRG neuron possesses one axon stemming from the cell body, which branches into two axons: a peripheral descending axon branch innervating peripheral targets and an ascending central branch that projects into the dorsal column of the spinal cord. Injuries of DRG axons have been widely used as an important model system to study the mechanisms that regulate axonal regeneration. Adult DRG neurons are among a few adult neurons known to regenerate robustly after injury. In addition, the peripheral and central branches of DRG neurons differ in their capacity to regenerate. The peripheral branches of the DRG neurons regenerate readily after peripheral nerve injury, whereas the central branches do not regrow after spinal cord injury. However, if peripheral axotomy occurs before the dorsal column injury (a process called conditioning lesion), central branches regain some ability to grow inside the spinal cord [3] . Clearly, understanding the molecular mechanisms that mediate peripheral axotomy-induced axon regeneration will help us develop strategies to enhance axon regeneration after central nervous system (CNS) injury. Moreover, the central branch shares the same CNS environment with descending corticospinal axons in the spinal cord, making the study relevant for CNS regeneration. To our knowledge, there is no approach currently available that directly targets mammalian adult DRG neurons for genetic manipulation via in vivo electroporation. Here we report a rapid and efficient approach to transfect adult DRG neurons in vivo with precise spatiotemporal control via electroporation. Using this approach, we have established three in vivo models of axon regeneration, in which DRG neurons can be genetically manipulated, including dorsal column transection, dorsal root rhizotomy and peripheral axotomy. By using the peripheral axotomy model, we performed a loss-of-function experiment by transfecting DRG neurons with small interfering RNAs (siRNAs) against c-jun to specifically deplete c-Jun. Our result provides ample evidence that c-Jun is required specifically during axon regeneration in the mature nervous system in vivo , and suggests a new perspective on the mechanism by which c-Jun regulates axon regeneration. Efficient delivery of genes into adult DRG neurons in vivo To transfect adult mouse DRGs (L4 and/or L5), DRGs were surgically exposed and injected with a plasmid DNA encoding enhanced green fluorescent protein (EGFP; Fig. 1a–c ), followed by electroporation with a pair of custom-made platinum tweezer-type electrodes ( Fig. 1d ). The survival rate of the electroporation experiments was nearly 100% ( ∼ 70 animals performed to date), and mice that recovered after the experiments showed no obvious signs of motor or sensory defects. To analyse the transfection results, electroporated DRGs were dissected out with their peripheral nerves and dorsal and ventral roots attached ( Fig. 2a ). When observed at 7 days after electroporation, EGFP-labelled neuronal cell bodies could be clearly detected in the ganglion ( Fig. 2b,c ). In addition, both the peripheral axons in the sciatic nerve and the central axons in the dorsal root stemming from the ganglion were also strongly labelled with EGFP ( Fig. 2b,c ). In contrast, EGFP-labelled axons were not found in the ventral root, which only contains axons from the spinal cord motor neurons ( Fig. 2b,c ). The labelled sensory axons were found all the way down to the nerve endings near the skin of the hind paw ( Fig. 2d ). By cross-sectioning the DRG and the sciatic nerve at site close to the ganglion, 384±56 (s.d.) EGFP-labelled axons ( n =3 mice) were observed, which represents about 5% of the total neurons in the DRG ( Fig. 2e,f ). This number of EGFP-expressing neurons, which is similar to that of the widely used Thy-1 GFP transgenic mice line M, is sufficient for quantitative analysis of axon regeneration. 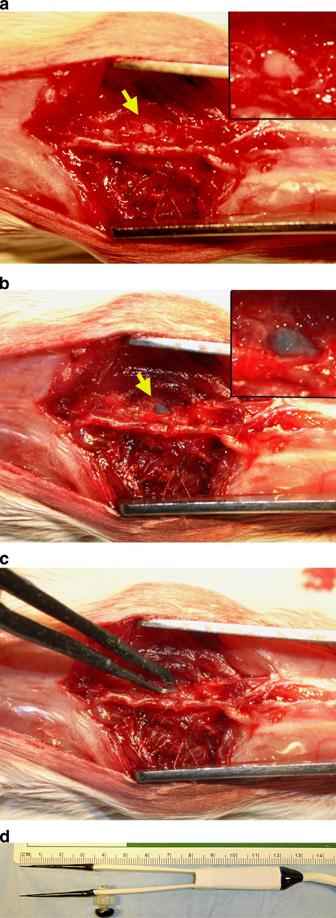Figure 1:In vivoelectroporation of adult mouse DRG neurons. (a) Image of a surgically exposed L4 DRG (yellow arrow and inset) on one side of the spinal cord. (b) Image of the surgically exposed DRG injected with a mixture of plasmid DNA and fast-green dye (yellow arrow and inset). (c) Image of the surgically exposed DRG being electroporated with the tweezer-like electrodes. (d) Image of the electrodes used in the study. Figure 1: In vivo electroporation of adult mouse DRG neurons. ( a ) Image of a surgically exposed L4 DRG (yellow arrow and inset) on one side of the spinal cord. ( b ) Image of the surgically exposed DRG injected with a mixture of plasmid DNA and fast-green dye (yellow arrow and inset). ( c ) Image of the surgically exposed DRG being electroporated with the tweezer-like electrodes. ( d ) Image of the electrodes used in the study. 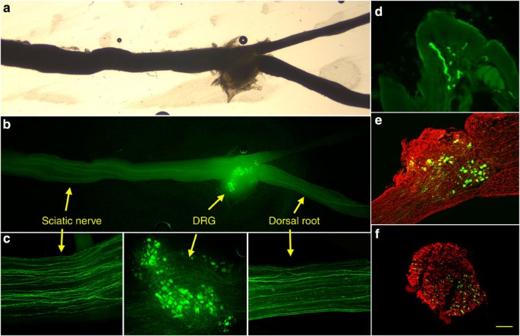Figure 2: Efficient gene transfection of adult DRG neurons. (a) An image of an electroporated DRG that was dissected out with its nerve attached at 7 days after electroporation. (b) A representative image of an electroporated DRG showing EGFP-labelled neuronal cell bodies in the ganglion and their axons in the sciatic nerve and the dorsal root. Note that no EGFP-labelled axons were observed in the ventral root. (c) Enlarged images for the indicated areas (yellow arrows) of panel b. (d) An image of EGFP-labelled axonal terminals in the hind paw skin sections. (e) Representative images of an EGFP-transfected DRG immunostained with the neuronal marker βIII tubulin (red). (f) Representative images of the peripheral nerve segment near the EGFP-transfected ganglion that was cross-sectioned and immunostained with βIII tubulin (red). Scale bars,a,b, 500 μm;c, 125 μm;d, 100 μm;e,f, 200 μm. Full size image Figure 2: Efficient gene transfection of adult DRG neurons. ( a ) An image of an electroporated DRG that was dissected out with its nerve attached at 7 days after electroporation. ( b ) A representative image of an electroporated DRG showing EGFP-labelled neuronal cell bodies in the ganglion and their axons in the sciatic nerve and the dorsal root. Note that no EGFP-labelled axons were observed in the ventral root. ( c ) Enlarged images for the indicated areas (yellow arrows) of panel b. ( d ) An image of EGFP-labelled axonal terminals in the hind paw skin sections. ( e ) Representative images of an EGFP-transfected DRG immunostained with the neuronal marker βIII tubulin (red). ( f ) Representative images of the peripheral nerve segment near the EGFP-transfected ganglion that was cross-sectioned and immunostained with βIII tubulin (red). Scale bars, a , b , 500 μm; c , 125 μm; d , 100 μm; e , f , 200 μm. Full size image When observed at 7 days after electroporation, EGFP expression was also detected in non-neuronal cells, in particular, at the proximal nerve segment close to the ganglion. These non-neuronal cells are S100 positive with tube-like morphology, satisfying the criteria for Schwann cells ( Fig. 3a ). Immunostaining with the antibody against NeuN, a neuronal marker, revealed that 43.5±3.5% (s.d.) of all EGFP-positive cells ( n =3, independent experiments) were neurons, indicating that electroporation had no preference for any specific cell types. General histological examination with haematoxylin and eosin staining did not reveal any observable signs of tissue damage or cell abnormality ( Fig. 3b ), showing that injection or electroporation per se did not cause any obvious cell death. Moreover, electroporation of DRGs did not induce caspase-3 activation, a widely used marker of apoptosis. In contrast, injection of DRGs with staurosporine, a reagent known to induce apoptosis [4] , resulted in strong staining of the active caspase-3 ( Fig. 3c,d ). Western blot analysis of the whole DRG lysate also confirmed that caspase-3 was not activated by electroporation ( Fig. 3e ), indicating that electroporation procedure per se did not induce cell apoptosis in DRGs. 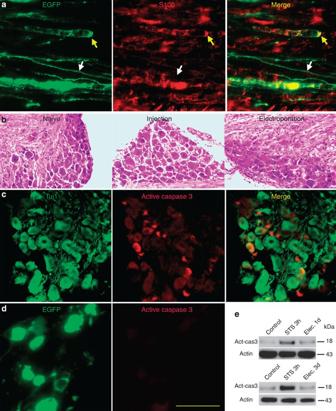Figure 3: Effects ofin vivoelectroporation. (a) Images of an area close to the ganglion transfected with EGFP. Note that both EGFP-positive axons and non-neuronal cells were identified, showing thatin vivoelectroporation of dorsal root ganglion (DRG) targets both neurons and non-neuronal cells. The white arrow indicates an axon labelled with EGFP. The yellow arrow indicates an EGFP-positive cell that is also positive for S100, the marker for Schwann cells. (b) Haematoxylin and eosin staining showing that neither plasmid injection nor electroporation had any detectable effects on the general histology of the DRG. (c) Representative immunostaining of the DRG injected with staurosporine. At 3 h after staurosporin injection, DRG was fixed and immunostained for active caspase-3 (red) and a neuronal marker Tuj1 (green). (d) Representative immunostaining of the DRG electroporated with EGFP. At 3 days after electroporation, DRG was fixed and immunostained for active caspase-3 (red). Note that electroporation of the DRG with EGFP caused no obvious apoptosis, indicated by the lack of active caspase-3 staining. (e) Representative immunoblots showing that the level of active caspase-3 (Act-cas3) in the DRG was not affected by electroporation (Elec.) when the DRG was subjected to western blot analysis at 1 day (Elec. 1d) or 3 days (Elec. 3d) after electroporation. By contrast, injection of staurosporine (STS) for 3 h increased the level of active caspase-3. Scale bars,a,b, 160 μm;c,d, 100 μm. Figure 3: Effects of in vivo electroporation. ( a ) Images of an area close to the ganglion transfected with EGFP. Note that both EGFP-positive axons and non-neuronal cells were identified, showing that in vivo electroporation of dorsal root ganglion (DRG) targets both neurons and non-neuronal cells. The white arrow indicates an axon labelled with EGFP. The yellow arrow indicates an EGFP-positive cell that is also positive for S100, the marker for Schwann cells. ( b ) Haematoxylin and eosin staining showing that neither plasmid injection nor electroporation had any detectable effects on the general histology of the DRG. ( c ) Representative immunostaining of the DRG injected with staurosporine. At 3 h after staurosporin injection, DRG was fixed and immunostained for active caspase-3 (red) and a neuronal marker Tuj1 (green). ( d ) Representative immunostaining of the DRG electroporated with EGFP. At 3 days after electroporation, DRG was fixed and immunostained for active caspase-3 (red). Note that electroporation of the DRG with EGFP caused no obvious apoptosis, indicated by the lack of active caspase-3 staining. ( e ) Representative immunoblots showing that the level of active caspase-3 (Act-cas3) in the DRG was not affected by electroporation (Elec.) when the DRG was subjected to western blot analysis at 1 day (Elec. 1d) or 3 days (Elec. 3d) after electroporation. By contrast, injection of staurosporine (STS) for 3 h increased the level of active caspase-3. Scale bars, a , b , 160 μm; c , d , 100 μm. Full size image When plasmids encoding EGFP and monomeric red fluorescent protein (mRFP) were mixed at a 1:1 ratio and co-transfected into the same DRG, most neurons expressed both EGFP and mRFP when observed at 7 days after electroporation ( Fig. 4a,b ). Co-transfection rate (% of EGFP-positive neurons also expressing mRFP) was 88.6±4.3% (s.d. ; n =3 mice). However, when L4 and L5 were electroporated with different plasmids (EGFP in L4 and mRFP in L5), axons labelled with EGFP and mRFP formed spatially separated bundles in the sciatic nerve ( Fig. 4c ). Strong expression of EGFP and mRFP in DRG neurons could be detected for at least 4 weeks. Together, these results indicate that in vivo electroporation enables delivery of genes into adult sensory neurons in an efficient and reproducible manner. 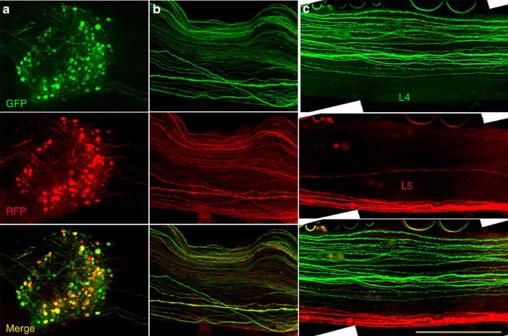Figure 4: Expression of multiple genes in DRG neurons. (a) The representative image of a DRG that was co-transfected with EGFP and mRFP. Most DRG neurons coexpressed EGFP and mRFP in their cell bodies. (b) The representative image of axons in the sciatic nerve coexpressing EGFP and mRFP. (c) The representative image of the sciatic nerve, which includes axons from L4 and L5 DRGs that were electroporated with EGFP and mRrP plasmids, respectively. Note that axons labelled with EGFP or mRFP were spatially separated in the same sciatic nerve (merged panel). Scale bars,a,b, 1,000 μm;c, 500 μm. Figure 4: Expression of multiple genes in DRG neurons. ( a ) The representative image of a DRG that was co-transfected with EGFP and mRFP. Most DRG neurons coexpressed EGFP and mRFP in their cell bodies. ( b ) The representative image of axons in the sciatic nerve coexpressing EGFP and mRFP. ( c ) The representative image of the sciatic nerve, which includes axons from L4 and L5 DRGs that were electroporated with EGFP and mRrP plasmids, respectively. Note that axons labelled with EGFP or mRFP were spatially separated in the same sciatic nerve (merged panel). Scale bars, a , b , 1,000 μm; c , 500 μm. Full size image Applying in vivo electroporation to access axon regeneration Adult sensory neurons have been widely used to study axon regeneration after peripheral or spinal cord injuries. Here we have applied the newly developed in vivo electroporation technique to assess axon regeneration by combining in vivo electroporation with well-established in vivo models of axon regeneration. The central branches of sensory axons enter the spinal cord through the dorsal root entry zone (DREZ), which borders the permissive environment in the peripheral nervous system and the inhibitory terrain in the CNS. CNS inhibitory molecules, especially the glial cell-derived chondroitin sulphate proteoglycans, are concentrated at the DREZ and prevent regenerating dorsal root axons from crossing the DREZ and re-entering the spinal cord [5] . As a result, axon growth across the DREZ after a dorsal root injury (rhizotomy) has been widely used to study axon regeneration over the inhibitory CNS environment [6] . At 7 days after in vivo electroporation, we found that dorsal root axons from control mice were clearly labelled with EGFP and entered the dorsal column through the DREZ ( Fig. 5a–e ). By contrast, when the dorsal root was crushed, regenerating axons stopped abruptly at DREZ ( Fig. 5f–h ) along the presumable border between the dorsal root and the spinal cord. No EGFP-positive axons were observed beyond this border. These results indicate that axon regeneration across the DREZ can be readily studied after in vivo electroporation of adult DRG neurons with selected plasmids/siRNAs. 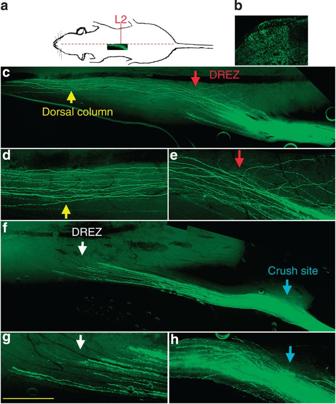Figure 5: Establishment of anin vivomodel of axon regeneration across the dorsal root entry zone. (a) Axons of L4 DRG enter the spinal cord at about the L2 level of the vertebrate. (b) Spinal cord cross-section above the L2 level at 7 days afterin vivoelectroporation of L4 DRG. Note that EGFP-labelled axons were detected in the spinal cord. (c) A representative image from a control mouse transfected with EGFP byin vivoelectroporation of L4 DRG. Note that EGFP-labelled dorsal root axons entered the spinal cord dorsal column. (d) Higher magnification image of the indicated areas in panel c (yellow arrow) for the dorsal column. (e) Higher magnification image of the indicated areas in panel c (red arrow) for the DREZ. (f) A representative image from a mouse that was injured by crushing in the middle of the dorsal root (cyan arrow). At 2 weeks after the crush, EGFP-labelled dorsal root axons regenerated within the dorsal root until they encountered the DREZ, where they stopped abruptly (white arrow). (g) Higher magnification image of the indicated areas in panel f (white arrow) for the DREZ. (h) Higher magnification image of the indicated areas in panel f (cyan arrow) for the crush site in the dorsal root. Scale bars,b,d,e,g,h, 400 μm;c,f, 1,000 μm. Figure 5: Establishment of an in vivo model of axon regeneration across the dorsal root entry zone. ( a ) Axons of L4 DRG enter the spinal cord at about the L2 level of the vertebrate. ( b ) Spinal cord cross-section above the L2 level at 7 days after in vivo electroporation of L4 DRG. Note that EGFP-labelled axons were detected in the spinal cord. ( c ) A representative image from a control mouse transfected with EGFP by in vivo electroporation of L4 DRG. Note that EGFP-labelled dorsal root axons entered the spinal cord dorsal column. ( d ) Higher magnification image of the indicated areas in panel c (yellow arrow) for the dorsal column. ( e ) Higher magnification image of the indicated areas in panel c (red arrow) for the DREZ. ( f ) A representative image from a mouse that was injured by crushing in the middle of the dorsal root (cyan arrow). At 2 weeks after the crush, EGFP-labelled dorsal root axons regenerated within the dorsal root until they encountered the DREZ, where they stopped abruptly (white arrow). ( g ) Higher magnification image of the indicated areas in panel f (white arrow) for the DREZ. ( h ) Higher magnification image of the indicated areas in panel f (cyan arrow) for the crush site in the dorsal root. Scale bars, b , d , e , g , h , 400 μm; c , f , 1,000 μm. Full size image Another widely used axon regeneration model is axon regeneration of sensory neurons in the spinal cord after a dorsal column transection. Under control condition, sensory axons in the dorsal column cannot regenerate beyond the injury site due to several factors, including the presence of multiple myelin-based CNS inhibitors and components in the glial scar [3] . In this study, we performed dorsal column transection at 7 days after in vivo electroporation and examined axon regeneration at 2 weeks after the transection ( Fig. 6a ). In some cases after nerve injury, we observed axon sprouting from axons labelled with EGFP after dorsal column transection, similar to that occurred in peripheral axons after the peripheral axotomy ( Fig. 6b ). Under the control condition, EGFP-labelled dorsal column axons failed to enter or grow beyond the lesion site ( Fig. 6c,d ), consistent with the previous studies using retrograde dye labelling [3] . A unique feature of the adult sensory axon regeneration is that axotomy of the peripheral branches of DRG neurons before the spinal cord injury can markedly promote the regeneration of the dorsal column axons, a phenomenon called the conditioning lesion effect [3] . Therefore, we next tested if the conditioning lesion effect could be reproduced in our in vivo electroporation model. When the sciatic nerve was lesioned at the same time as in vivo electroporation and the dorsal column was transected 7 days later, regeneration of EGFP-labelled dorsal column axons was markedly improved ( Fig. 5e,f ). Many axons entered the lesion site and some of them grew well beyond it when observed at 2 weeks after the dorsal column transection. Therefore, by combining in vivo electroporation with the spinal cord injury model, it is possible to genetically manipulate DRG neurons and investigate molecular and/or cellular mechanisms of axon regeneration. 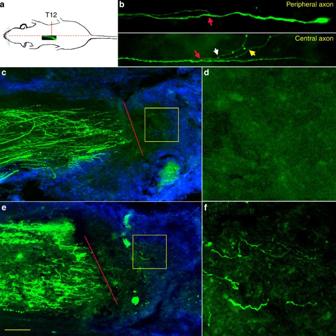Figure 6: Establishment of anin vivomodel of dorsal column axon regeneration. (a) Afterin vivoelectroporation of the L4 DRG, a dorsal column transection was performed at about the T12 level of the vertebrate. (b) The top panel shows peripheral axon sprouting in the peripheral nerve at a single axon level after a peripheral axotomy. Red arrow indicates the branching point. The bottom panel shows sprouting of the DRG central axon inside the spinal cord after dorsal column transection. Red, white and yellow arrow indicates primary, secondary and tertiary branching points, respectively. (c) A representative image from a control mouse showing that transection of the dorsal column axons (red line indicates the injury site) resulted in no axon regeneration into or beyond the injury site when observed at 2 weeks after the injury. (d) An enlarged image of the yellow square in panel c. (e) A representative image from a mouse that was subjected to peripheral axotomy (conditioning lesion) 1 week before the dorsal column transection (red line indicates the injury site). Note that many EGFP-labelled axons grew into and beyond the lesion site. (f) An enlarged image of the yellow square in panele. Scale bars,b,d,f, 50 μm;c,e, 200 μm. Figure 6: Establishment of an in vivo model of dorsal column axon regeneration. ( a ) After in vivo electroporation of the L4 DRG, a dorsal column transection was performed at about the T12 level of the vertebrate. ( b ) The top panel shows peripheral axon sprouting in the peripheral nerve at a single axon level after a peripheral axotomy. Red arrow indicates the branching point. The bottom panel shows sprouting of the DRG central axon inside the spinal cord after dorsal column transection. Red, white and yellow arrow indicates primary, secondary and tertiary branching points, respectively. ( c ) A representative image from a control mouse showing that transection of the dorsal column axons (red line indicates the injury site) resulted in no axon regeneration into or beyond the injury site when observed at 2 weeks after the injury. ( d ) An enlarged image of the yellow square in panel c. ( e ) A representative image from a mouse that was subjected to peripheral axotomy (conditioning lesion) 1 week before the dorsal column transection (red line indicates the injury site). Note that many EGFP-labelled axons grew into and beyond the lesion site. ( f ) An enlarged image of the yellow square in panel e . Scale bars, b , d , f , 50 μm; c , e , 200 μm. Full size image Finally, we applied the in vivo electroporation method to study peripheral axon regeneration. To this end, sciatic nerves were crushed at 3 days after in vivo electroporation, and axon regeneration was analysed 4 days later by directly measuring the length between tips of regenerating axons and the crush site. Under control condition, axons regenerated at a rate of 1.36±0.4 (s.d.) mm per day ( n =5 mice; Fig. 7 ), consistent with previous studies from the Thy-1 YFP mice [7] , [8] . This result indicates that electroporation per se does not affect the axon growth ability of adult DRG neurons. In Thy-1 YFP mice, some YFP remains in the distal nerve stump a few days after the nerve crush due to Wallerian degeneration. These fluorescently labelled debris often interfere with the definitive identification of regenerating axons [9] , hindering quantitative analysis of axon regeneration. Here in our study, ectopically expressed EGFP was rarely detected beyond the nerve crush site when observed at 3 days after electroporation. Therefore, identification of regenerating axon tips was not obscured by debris from degenerating axons. Together, in vivo electroporation of adult DRG neurons can be an effective tool to genetically manipulate sensory neurons for studying axon regeneration after CNS or peripheral nervous system injuries. 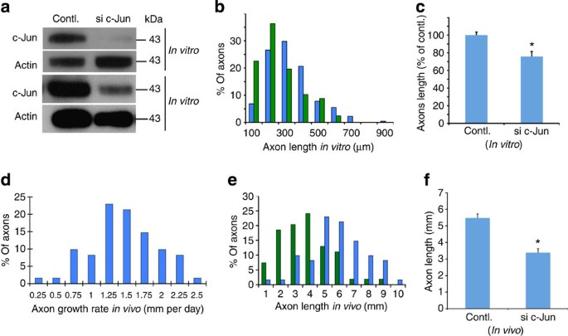Figure 7: Specific knock down of c-Jun in adult sensory neurons inhibits axotomy-induced axon regeneration. (a) Representative immunoblots using adult DRGs that were transfected with control or a mixture of four different siRNAs againstc-jun(ON-TARGETplus, Dharmacon) eitherin vitroorin vivo. Note that c-Jun was efficiently knocked down bothin vitroandin vivo. (b) Distribution of axon lengths of control and si-c-jun-transfected neurons. Shown are distributions of axon lengths from control (blue) and si-c-jun-transfected neurons (green). (c) Average axon lengths from control (n=5 mice) and si-c-jun-transfected neurons (n=5 mice). *P=0.022 (two-tailed Student'st-test) compared with control. (d) Distribution ofin vivoaxon regeneration rates of EGFP-transfected neurons after sciatic nerve crush under control condition. A total of 71 axons pooled from five mice were included in the analysis. (e) Distribution of axon regeneration lengths of control and si-c-jun-transfected mice when analysed at 4 days after nerve crush. A total of 142 axons pooled from ten mice were included in the analysis for control and si-c-Jun (71 axons from five mice for control; 71 axons from five mice for si-c-Jun). (f) Average axon lengths of control (n=5 mice) and si-c-jun-transfected neurons (n=5 mice) when analysed at 4 days after nerve crush. *P<0.00001 (two-tailed Student'st-test) compared with control. Comparison is made between animals. Error bars indicate standard error of the mean. Figure 7: Specific knock down of c-Jun in adult sensory neurons inhibits axotomy-induced axon regeneration. ( a ) Representative immunoblots using adult DRGs that were transfected with control or a mixture of four different siRNAs against c-jun (ON-TARGET plus , Dharmacon) either in vitro or in vivo . Note that c-Jun was efficiently knocked down both in vitro and in vivo . ( b ) Distribution of axon lengths of control and si- c-jun -transfected neurons. Shown are distributions of axon lengths from control (blue) and si- c-jun -transfected neurons (green). ( c ) Average axon lengths from control ( n =5 mice) and si- c-jun- transfected neurons ( n =5 mice). * P =0.022 (two-tailed Student's t -test) compared with control. ( d ) Distribution of in vivo axon regeneration rates of EGFP-transfected neurons after sciatic nerve crush under control condition. A total of 71 axons pooled from five mice were included in the analysis. ( e ) Distribution of axon regeneration lengths of control and si- c-jun -transfected mice when analysed at 4 days after nerve crush. A total of 142 axons pooled from ten mice were included in the analysis for control and si-c-Jun (71 axons from five mice for control; 71 axons from five mice for si-c-Jun). ( f ) Average axon lengths of control ( n =5 mice) and si- c-jun -transfected neurons ( n =5 mice) when analysed at 4 days after nerve crush. * P <0.00001 (two-tailed Student's t- test) compared with control. Comparison is made between animals. Error bars indicate standard error of the mean. Full size image Axon regeneration is impaired by acute depletion of c-Jun Robust axon regeneration of DRG neurons after peripheral axotomy is attributed to the activation of a group of regeneration-associated genes (RAGs) [10] , such as c-Jun, which is a component of the AP-1 transcription factor complex. c-Jun is upregulated and coexpressed with the growth-associated protein GAP-43 in adult DRG neurons after axotomy for several weeks during peripheral regeneration [11] . The in vivo role of c-Jun in axon regeneration has been examined by conditional knockout of c-Jun in facial motor neurons using nestin-Cre-mediated recombination [12] , which deletes c-Jun in neural progenitors both in CNS and peripheral nervous system during development. Although no apparent developmental abnormality was observed in the nervous system of c-Jun conditional knockout mice, it is still possible that compensatory responses that might have taken place during development in the c-Jun knockout mice contributes to the regeneration defect observed in adult animals [13] . In this study, we investigated whether and how acute depletion of c-Jun in sensory neurons of a mature animal affects axon regeneration. To deplete endogenous c-Jun, we used a group of four siRNAs targeting different regions in c-jun (si-c-Jun), which are designed to minimize the off-target effects (ON-TARGET plus , Thermo Scientific Dharmacon). Transfection of this pool of siRNAs dramatically reduced c-Jun level in both cultured adult DRG neurons and in vivo ( Fig. 7a ). To examine if acute depletion of c-Jun affected axon regeneration in vitro , adult DRG neurons were dissociated and transfected with si-c-Jun, and cultured for 3 days to allow depletion of endogenous c-Jun. When these neurons were replated to allow axon regrowth, regenerative axon growth from c-Jun-depleted neurons was significantly impaired as compared with control neurons ( Fig. 7b,c ). To examine if these results can be recapitulated in vivo , we performed in vivo electroporation of DRG neurons with si-c-Jun and EGFP. Si-c-Jun also markedly knocked down c-Jun in DRGs in vivo ( Fig. 7a ). When sciatic nerves of the electroporated mice were crushed at 3 days after electroporation, and axon regeneration was examined 4 days later, sensory axons from c-Jun-depleted neurons displayed significantly impaired axon regeneration in vivo compared with control neurons ( Fig. 7e,f ). From the EGFP signals of the transfected neurons we noticed that, under control condition, most regenerating axons had enlarged growing tips ( Fig. 8a,c ), indicative of actively growing growth cones. In contrast, axons from neurons transfected with si-c-Jun showed obvious thinning of distal axonal tips ( Fig. 8b,c ). The reduction in growth cone size by depletion of c-Jun was confirmed by quantification ( Fig. 8d,e ). Such distal axon thinning is indicative of atrophic growth cones, which is different from the retraction bulbs that form when regenerating axons encounter inhibitory molecules [14] . These results indicate that c-Jun regulates axon assembly through a mechanism that modulates growth cone morphology. 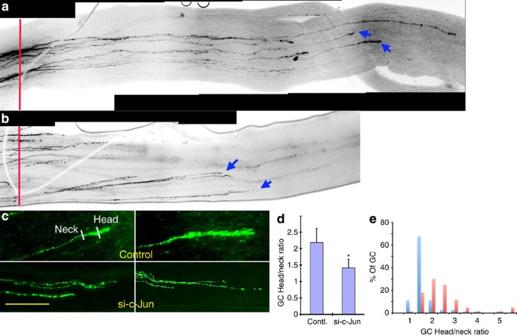Figure 8: Knock down of c-Jun affects growth cone morphologies of regenerating axonsin vivo. (a) A representative image of control regenerating axons growing from L4 DRG that was transfected with EGFP. Red line indicates the crush site. Blue arrows indicate distal ends (growth cones, GCs) of regenerating axons. (b) A representative image of regenerating axons from L4 DRG that was transfected with a mixture ofc-junsiRNA and EGFP. Red line indicates the crush site. Blue arrows are distal ends (growth cones) of regenerating axons. (c) Enlarged images of growth cones from panelsaandb(blue arrows). Control axons had enlarged distal ends, indicative of actively advancing growth cones, whereas c-Jun-depleted axons had much thinner tips, indicative of dystrophic growth cones. (d) Quantification of the size of the distal axon ends. For quantification, the width of the enlarged portion of the distal axon (head) was measured and is presented as a ratio with respect to the width of the adjacent axon shaft (neck). Depletion of c-Jun significantly reduced the head/neck ratio. *P<0.00001 (two-tailed Student'st-test) compared with control (n=5 mice for each group). Comparison is made between animals. (e) Distribution of the head/neck ratios of control and si-c-jun-transfected neurons shows that the majority of control axons (∼78%) had the head/neck ratio higher than 2, whereas most axons lacking c-Jun (∼79%) had the ratio less than 2. A total of 142 axons pooled from ten mice were included in the analysis for control and si-c-Jun (71 axons from five mice for control; 71 axons from five mice for si-c-Jun). The same axons were used for analysing both axon growth (7b–f) and growth cone morphology (8d,e). Scale bars,a,b, 1,000 μm;c, 200 μm. Error bars indicate standard error of the mean. Figure 8: Knock down of c-Jun affects growth cone morphologies of regenerating axons in vivo . ( a ) A representative image of control regenerating axons growing from L4 DRG that was transfected with EGFP. Red line indicates the crush site. Blue arrows indicate distal ends (growth cones, GCs) of regenerating axons. ( b ) A representative image of regenerating axons from L4 DRG that was transfected with a mixture of c-jun siRNA and EGFP. Red line indicates the crush site. Blue arrows are distal ends (growth cones) of regenerating axons. ( c ) Enlarged images of growth cones from panels a and b (blue arrows). Control axons had enlarged distal ends, indicative of actively advancing growth cones, whereas c-Jun-depleted axons had much thinner tips, indicative of dystrophic growth cones. ( d ) Quantification of the size of the distal axon ends. For quantification, the width of the enlarged portion of the distal axon (head) was measured and is presented as a ratio with respect to the width of the adjacent axon shaft (neck). Depletion of c-Jun significantly reduced the head/neck ratio. * P <0.00001 (two-tailed Student's t -test) compared with control ( n =5 mice for each group). Comparison is made between animals. ( e ) Distribution of the head/neck ratios of control and si- c-jun -transfected neurons shows that the majority of control axons ( ∼ 78%) had the head/neck ratio higher than 2, whereas most axons lacking c-Jun ( ∼ 79%) had the ratio less than 2. A total of 142 axons pooled from ten mice were included in the analysis for control and si-c-Jun (71 axons from five mice for control; 71 axons from five mice for si-c-Jun). The same axons were used for analysing both axon growth ( 7b–f ) and growth cone morphology ( 8d,e ). Scale bars, a , b , 1,000 μm; c , 200 μm. Error bars indicate standard error of the mean. Full size image In summary, our study validates in vivo electroporation as a useful tool to genetically dissect the roles of RAGs in axon regeneration. In addition, it provides strong evidence for the in vivo role of c-Jun, specifically during axon regeneration, and suggests a potential cellular mechanism by which c-Jun controls axon regeneration. In vivo electroporation of adult sensory neurons established in this study provides a powerful tool to study axon regeneration in vivo . First, by electroporating different constructs into different DRGs in the same animal ( Fig. 3 ), it is possible to perform mosaic analysis to study gene function in axon regeneration. Because both control and experimental groups can be included in the same animal, the variability among different animals is also minimized. Second, because transfected genes start to be expressed within a few hours after electroporation, it will allow precise temporal manipulation of gene expression to study axon regeneration, which cannot be achieved by either inducible transgenic technique or viral-mediated genetic approach. With the newly developed technique, it is now possible to regulate gene expression at or near the time of neural injury in adult mice and directly investigate the possible role of candidate genes specifically during regeneration without alterations in other compensatory responses that might take place during embryogenesis and postnatal stages. Third, with the availability of expression constructs or siRNA/short hairpin RNA for most genes, this approach will allow genetic studies of axon regeneration in vivo at much higher throughput compared with the traditional transgenic approach. Although viral-mediated transfection of DRG neurons can be achieved through injection at the peripheral nerve without complicated surgery, the preparation and purification of virus for each gene of interest can be more time consuming as compared with the surgery, which typically can be completed within 2 h (including the electroporation) with nearly 100% survival rate. Moreover, with electroporation, multiple constructs can be readily co-transfected into the same neuron, thus allowing modulation of multiple genes simultaneously. This approach is of particular importance in investigating the role of a signalling pathway(s) and defining upstream–downstream relationships of molecules of interest in a certain pathway. Fourth, by using EGFP or EGFP-fused proteins, axon regeneration can be directly analysed without retrograde dye labelling, which sometimes may cause false labelling and affect interpretation of the study [15] , [16] . Finally, by electroporating and expressing the plasmid encoding the recombinase Cre in animals carrying floxed genes, this approach will also allow gene knockout in adult sensory neurons with precise temporal control. Taken together, the in vivo electroporation technique that we introduce in the present study opens the possibility of investigating axon regeneration in a way that was not previously possible. One potential pitfall of this technique is that electroporation targets both neurons and non-neuronal cells in the DRG, which may complicate the interpretation of the obtained results. However, combination of neuron-specific promoters should solve this problem and allow specific manipulation of gene expression in neurons. In addition, this method might not be suitable for behaviour studies because the transfection efficiency of electroporation is relatively low as compared with transgenic approach or viral-mediated gene delivery. Peripheral axotomy of DRG axons is well known to activate the intrinsic axon growth ability via inducing the expression of RAGs [10] . This study provides strong and novel evidence about the in vivo role of c-Jun in the regulation of axon regeneration, although a previous study showed that c-Jun is involved in axon regeneration by using conditional knock out approaches [12] . First, by direct in vivo electroporation of adult DRG neurons, c-Jun was specifically and acutely deleted in neurons of a mature animal, whereas the conditional nestin-Cre knockout approach targeted neural progenitors during development. Second, after axotomy c-Jun is upregulated not only in neurons but also in non-neuronal cells, such as Schwann cells [17] , in which c-Jun controls Schwann cell proliferation/differentiation and myelination [18] . Because nestin-Cre-mediated recombination also targets Schwann cells in the nerve, which are known to be important for axon regeneration, it is possible that depletion of c-Jun in the Schwann cells at the injury site may have contributed to the reduced facial nerve regeneration. In this study, although Schwann cells close to the neuronal soma were transfected ( Fig. 3 ), Schwann cells at the injury site were unaffected. Thus, our results indicate stronger evidence about the specific role of neuronal c-Jun in axon regeneration. Finally, in our study we could directly examine how c-Jun knockdown affected the morphologies of regenerating axons ( Fig. 8 ), which suggests potential novel cellular mechanisms by which c-Jun controls axon regeneration. In addition to c-jun , many genetic profiling studies have identified hundreds of other RAGs upon peripheral axotomy. Illustrating the roles of these RAGs in axon regeneration will not only help us understand how peripheral axotomy induces the robust regeneration in adult DRG neurons, but also identify potential targets to enhance the regeneration ability of adult CNS neurons. However, to date, very few in vivo studies have reported the functions of these RAGs in axon regeneration, presumably due to the difficulty to genetically manipulate these genes in vivo , specifically in adult neurons. By combining in vitro cell culture and the in vivo model established in this study, higher-throughput screen of the roles of these RAGs in axon regeneration in vivo is now possible. Importantly, the dorsal column regeneration model can be used to investigate if a particular RAG identified in the screen can promote dorsal column axon regeneration in the spinal cord. Furthermore, the acute genetic manipulation of adult DRG neurons may provide an alternative approach to study the roles of CNS myelin-based inhibitors in axon regeneration after spinal cord injuries. The current studies using the conventional knockout approach have generated conflicting results [19] , [20] , [21] , [22] , [23] , [24] , possibly due to the compensatory genetic changes of other CNS inhibitory molecules [25] . In summary, our study presented here not only provides a valuable tool to manipulate gene expression in adult sensory neurons in vivo , but also establish a powerful in vivo model to study axon regeneration. Plasmids and antibodies The plasmids used in the study were pCMV–EGFP–N1 (Clontech) and pCMV–mRFP–N1 (Clontech). The siRNAs against c-jun (ON-TARGET plus ) were from Thermo Scientific Dharmacon. The βIII tubulin antibody (TUJ1) was from Sigma-Aldrich. The antibodies against c-Jun and cleaved caspase-3 were from Cell Signaling Technology. The NeuN antibody was from Millipore and S100 antibody was from Dako. In vivo electroporation Eight- to ten-week-old female CF-1 mice (weighing from 30 to 35 g) were purchased from Charles River Laboratories and housed in the university animal facility. All experiments involving animals were performed in accordance with the animal protocol approved by the Institutional Animal Care and Use Committee of the Johns Hopkins University. The mice were anaesthetized with intra-peritoneal injection of a mixture of katamine (100 mg kg −1 ) and xylazine (10 mg kg −1 ). A 3-cm-long skin incision was made aseptically at the midline of the lower back. The overlaying muscles were dissected and removed from the L4–L5 spinous processes. To expose the L4 or L5 DRG, a small dorsolateral laminectomy was performed by removing the processus accessorius and part of the processus transverses. For DNA injection, 10-cm capillary glass tubes (Sutter Instrument) were pulled by using a micropipette puller model 720 (David KOPF Instrument; heater, 13.6; solenoid: 3). The tips of pulled-out capillary glass pipettes were pinched with forceps to generate about 80 μm external diameter pipettes. Solution of DNA plasmids (1.0 μl) or siRNAs was gradually injected into the DRG using a Picospritzer II (Parker Ins. ; pressure, 30 psi; duration: 8 ms). The plasmid concentration was 2–3 μg μl −1 and the siRNAs were used at 50 pMol μl −1 . DNA plasmids were dissolved in distilled, deionized water and siRNAs were dissolved in the siRNA buffer provided by the manufacturer (Dharmacon). Electroporation was performed immediately after the injection using a custom-made tweezer-like electrode (Ø1.2 mm) and a BTX ECM830 Electro Square Porator (five 15 ms pulses at 35 V with 950 ms interval). The gap between electrode was 1.2±0.2 mm. After electroporation, the wound was closed and the mice were allowed to recover. Spinal cord and nerve injuries For the dorsal root crush, the mice were anaesthetized as described above. A small laminectomy was performed at the L2–L3 level. After opening the dura, the EGFP-labelled dorsal root from the L4 DRG was carefully exposed using a fine glass hook. The nerve was then crushed for 30 s using a pair of fine forceps. For the dorsal column lesion, a dorsal laminectomy at T12 level was performed to expose the spinal cord. A bilateral dorsal hemisection was then performed with ophthalmic micro-scissors, resulting in a complete cut of the dorsal column. For the peripheral nerve conditioning lesion experiment, the sciatic nerve was exposed and transected at the mid-thigh level with micro-scissors. For the peripheral nerve regeneration experiment, the sciatic nerve was exposed at the sciatic notch by a small incision. The nerve was then crushed with a pair of fine forceps and the crush site was marked with a size 10-0 nylon epineural suture. After surgeries, the wound was closed and the mice were allowed to recover. Tissue preparation and immunostaining The mice were terminally anaesthetized and transcardially perfused with phosphate-buffered saline (PBS, pH 7.4), followed by ice-cold 4% paraformaldehyde (PFA) in PBS. The tissues of interest from the perfused animal were carefully dissected out and postfixed overnight in 4% PFA at 4 °C. DRGs with sciatic nerves attached or spinal cords with dorsal roots attached were whole mounted without sectioning. Some DRGs or spinal cords were cryoprotected in PBS containing 30% sucrose for 24 h at 4 °C, and embedded in optical cutting temperature compound (Sakura) on dry ice. Cryosections at 20 μm were cut on a cryostat and processed for either immunostaining or direct imaging. Sections of electroporated DRGs were immunostained with βIII tubulin antibody (TUJ1) to label neurons, S100 antibody to label Schwann cells or antibody against cleaved caspase-3 to label apoptotic cells. The secondary antibodies used were goat anti-mouse/rabbit Alexa Flour 488/568 (Invitrogen). Primary culture of mouse adult DRG neurons Adult DRG neurons were cultured as described previously [26] . Briefly, DRGs were dissected out and digested with collagenase A (1 mg ml −1 ) for 90 min, followed by trypsin-EDTA (0.05%) for 20 min at 37.0 °C. The digested DRGs were then washed three times with culture medium (MEM with L -glutamine, 1× penicillin/streptomycin and 5% fetal calf serum) and dissociated with a 1-ml pipette tip in culture medium. The dissociated neurons were centrifuged to remove the supernatant and resuspended in 80 μl of Amaxa electroporation buffer (for mouse neuron) with mixtures of siRNAs and the EGFP plasmid. The suspended cells were then transferred to a 2.0-mm cuvette and electroporated with the Amaxa Nucleofector apparatus. After electroporation, cells were immediately transferred to the desired volume of prewarmed culture medium and plated on culture dishes coated with poly- D -lysine (100 μg ml −1 ) and laminin (10 μg ml −1 ). After neurons fully attached to the substrates (4–6 h), the medium was changed to remove the remnant electroporation buffer. For in vitro axon growth assay, the transfected neurons were cultured for 3 days to allow knocking down of the endogenous proteins (c-Jun). The cells were then resuspended and replated. After overnight culture, the replated adult DRG neurons were fixed with 4% PFA and then stained with anti-β III tubulin antibody. Fluorescence imaging and axon growth quantification The images of the whole-mount tissues, the cryosections or the cultured cells were captured with an inverted light microscope (Zeiss Axiovert200, Carl Zeiss MicroImaging) equipped with epifluorescence optics and a charge-coupled device camera controlled by Axiovision software (Carl Zeiss MicroImaging). To quantify axon growth in vitro , the longest axon from each neuron (≥1 cell body diameter) was traced manually and the axon length was measured with the 'measure/curve' application of AxioVision 4.6 software (Carl Zeiss MicroImaging). For in vivo axon regeneration, every identifiable EGFP-labelled axon in the sciatic nerve was manually traced from the crush site to the distal growth cone to measure the axon length. To quantify the growth cone size of regenerating axons in the sciatic nerve, the width of the enlarged portion of the distal axon end (growth cone head) was measured, and its ratio with respect to the width of the immediate adjacent axon shaft (growth cone neck) was calculated. Western blot analysis For the in vitro knocking down experiment, dissociated adult DRG neurons were transfected with siRNAs against c-jun and cultured for 3 days. The cells were then lysed with the RIPA buffer and processed for western blot analysis. For the in vivo knocking down experiment, 3 days after in vivo electroporation of c-jun siRNAs, the DRG was dissected out and homogenized. The protein extracts were then processed for western blot. The protein level of c-Jun was detected with the rabbit anti-c-Jun antibody at 1:1,000 dilutions. Statistics Quantification data were presented as mean±s.e.m. (unless indicated as s.d.). Two-tailed Student's t- test with an α -level of 0.05 was used to determine the statistical significance between different experimental groups. How to cite this article: Saijilafu et al . Genetic dissection of axon regeneration via in vivo electroporation of adult mouse sensory neurons. Nat. Commun. 2:543 doi: 10.1038/ncomms1568 (2011).